Nitric oxide enhances Th9 cell differentiation and airway inflammation Th9 cells protect hosts against helminthic infection but also mediate allergic disease. Here we show that nitric oxide (NO) promotes Th9 cell polarization of murine and human CD4 + T cells. NO de-represses the tumour suppressor gene p53 via nitrosylation of Mdm2. NO also increases p53-mediated IL-2 production, STAT5 phosphorylation and IRF4 expression, all essential for Th9 polarization. NO also increases the expression of TGFβR and IL-4R, pivotal to Th9 polarization. OVA-sensitized mice treated with an NO donor developed more severe airway inflammation. Transferred Th9 cells induced airway inflammation, which was exacerbated by NO and blocked by anti-IL-9 antibody. Nos2 −/− mice had less Th9 cells and developed attenuated eosinophilia during OVA-induced airway inflammation compared with wild-type mice. Our data demonstrate that NO is an important endogenous inducer of Th9 cells and provide a hitherto unrecognized mechanism for NO-mediated airway inflammation via the expansion of Th9 cells. It is now generally accepted that CD4 + T cells are functionally divided into various subsets: Th1, Th2, Th17, Th9 and Tregs (regulatory T cells). Although plasticity among these subsets are frequently reported, these cells are mainly defined by the cytokines they produce together with their signature master transcription factors (reviewed in ref. 1 ). Th9 is the latest subset of Th cells defined by their production of interleukin (IL)-9 (refs 2 , 3 ), the transcription factors PU.1 (ref. 4 ) and interferon regulatory factor 4 (IRF4) (ref. 5 ), although these factors are not unique to Th9. IL-9 has been considered a classical type 2 cytokine, and is associated with the host defence against intestinal nematode infection and the development of allergic responses. Mice overexpressing IL-9 develop intestinal mastocytosis and are resistant to Trichuris muris infection [6] , [7] and administration of neutralizing anti-IL-9 antibody abrogated the worm expulsion [8] . Consistent with the characteristics of type 2 cytokines, overexpression of IL-9 in the lung led to spontaneous airway inflammation in mice [9] , [10] . Increased expression of IL-9 and its receptor were also found in the lungs of asthmatic patients [11] . Th9 cells as a source of IL-9 contribute to allergic inflammation [4] , [5] . In humans, allergic donors have substantially more circulating Th9 cells than non-allergic donors [12] . Th9 cells are generated in vitro by culturing naive CD4 + T cells with IL-4 and tumour growth factor-β (TGFβ) [2] , [3] , [13] . This pair of cytokines forms the basic environment for driving Th9 cells, the polarizing of which can be enhanced by the presence of IL-1 (refs 14 , 15 ), IL-2 (ref. 13 ) and IL-25 (ref. 16 ). We report here that nitric oxide (NO), a free radical, is a potent enhancer of Th9 polarization and maintenance. NO is a crucial mediator of a range of biological functions, including vascular relaxation, platelet aggregation, neurotransmission, tumoricidal and microbicidal activities, and immune regulation (reviewed in refs 17 , 18 , 19 , 20 ). NO is also associated with some of the most important immune pathologies, including rheumatoid arthritis, diabetes, systemic lupus erythematosus and septic shock. NO is derived from the guanidino nitrogen atom(s) and molecular oxygen in a reaction catalysed by three forms of NO synthase (NOS). The neuronal form (nNOS or NOS1) and endothelial form (eNOS or NOS3) produce physiological level of NO at steady state. The cytokine-inducible form (iNOS or NOS2) is activated by a number of immunological stimuli, including interferon-γ (IFNγ), tumour necrosis factor-α and LPS generated during infection, and catalyses high output of NO, which can be cytotoxic and kill intracellular pathogens. We have recently shown [21] that NO can suppress the proliferation and function of polarized murine and human Th17 cells via the downregulation of the expression of aryl hydrocarbon receptor that participates in the induction of Th17. We now show that, in contrast to its effect on Th17, NO markedly enhances the polarization and function of Th9 cells. NO does so by elevating the expression of p53, which in turn increases the production of IL-2 and activates the downstream events including phosphorylation of signal transducer and activator of transcription 5 (STAT5) and the expression of IRF4. In vivo , administration of an NO donor increases airway inflammation, whereas Nos2 -deficiency reduces Th9 cell development and allergic reaction. Our data demonstrate a hitherto unrecognized NO function, and indicate that NO is an important endogenous inducer of Th9 responses and may have a key role in infectious and allergic diseases. NO inhibits Th17 but enhances Th9 differentiation We reported recently that NO selectively inhibits the differentiation of Th17 cells [21] . We then investigated the effect of NO on the expression of other genes during Th17 differentiation. CD4 + T cells were purified from the spleen and lymph nodes of naive BALB/c mice and cultured under a Th17 polarizing conditions (anti-CD3 antibodies+IL-6, TGFβ, IL-1β, IL-23, anti-IFNγ, anti-IL-4 and mitomycin C-treated antigen-presenting cells, APCs) in the presence of 100 μM of NOC-18 (an NO donor) as described previously [21] . The cells were harvested 72 h after the culture (when all APCs had disappeared), and total RNA was extracted and subjected to microarray analysis. As expected, a vast array of messages was affected by the presence of NO ( Fig. 1a and Supplementary Fig. 1 ). Focusing on cytokines, Il17a message was clearly decreased but Il24, Il22, Il9 and Il2 mRNA were markedly upregulated ( Fig. 1a ). In this report, we elected to focus on IL-9. The enhancement of Il9 expression by NO was confirmed by quantitative PCR (qPCR) assay ( Fig. 1b ) and by enzyme-linked immunosorbent assay (ELISA) of the culture supernatants ( Fig. 1c ). Fluorescence-activated cell sorting (FACS) analysis demonstrated that decrease in the percentage of IL-17 + T cells was accompanied by an increase in the percentage of IL-9 + T cells and IL-17/IL-9 double-positive T cells ( Fig. 1d,e ). We then determined whether NO can influence the differentiation of Th17 and Th9 cells under the mixed polarization conditions for Th17 and Th9. CD4 + T cells were cultured for 4 days with plate-bounded anti-CD3 and soluble anti-CD28+IL-4, TGFβ, IL-6, IL-1β, IL-23 and anti-IFNγ (without APC) in the presence of NOC-18. These culture conditions resulted in a modest percentage of Th17 cells and a distinct population of Th9 cells. NO decreased the percentage of IL-17 + cells and enhanced the percentage of IL-9 + T cells without producing significant number of IL-17/IL-9 double-positive T cells ( Fig. 1f ). The differential effect of NO on Th17 and Th9 cell polarization was also reflected in the concentrations of IL-9 and IL-17 in the supernatants of these cultures ( Fig. 1g ). These results therefore demonstrate that NO inhibits Th17 development but enhances the differentiation of Th9 cells under Th17 and Th17/9 polarizing conditions. 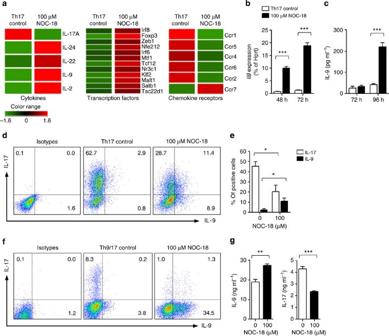Figure 1: NO inhibits Th17 but enhances Th9 development. Purified BALB/c CD4+T cells were cultured for 3 days under Th17 polarizing conditions (round-bottom 96-well plate with APC, αCD3, IL-6, TGFβ, IL-23, IL-1β, αIFNγ and αIL-4). NO donor (NOC-18) was added at the beginning of culture. (a) Microarray analysis of differential mRNA expression between cells cultured with or without NO. Full microarray information is provided inSupplementary Fig. 1and deposited in MIAME (E-MEXP-3959). (b)Il9mRNA was further quantified by qPCR. (c) IL-9 concentration in the supernatant was determined by ELISA. (d) IL-17- and IL-9-producing cells were analysed by FACS. Numbers in quadrants indicate percentage of cells and are summarized ine. (f) CD4+T cells were cultured under Th17/Th9 conditions (αCD3+IL-4, TGFβ, IL-6, IL-1β, IL-23 and anti-IFNγ)±NO. Percentage of cells producing IL-9 and IL-17 was determined by FACS. (g) IL-9 and IL-17 concentrations in the culture supernatant was assayed by ELISA. Data are representative of at least three independent experiments; Mean±s.e.m.,n=3; *P<0.05, **P<0.01, ***P<0.001 using a two-way analysis of variance (b,c,e) or a two-tailed unpaired Student’st-test (g). Hprt, hypoxanthine-guanine phosphoribosyltransferase. Figure 1: NO inhibits Th17 but enhances Th9 development. Purified BALB/c CD4 + T cells were cultured for 3 days under Th17 polarizing conditions (round-bottom 96-well plate with APC, αCD3, IL-6, TGFβ, IL-23, IL-1β, αIFNγ and αIL-4). NO donor (NOC-18) was added at the beginning of culture. ( a ) Microarray analysis of differential mRNA expression between cells cultured with or without NO. Full microarray information is provided in Supplementary Fig. 1 and deposited in MIAME (E-MEXP-3959). ( b ) Il9 mRNA was further quantified by qPCR. ( c ) IL-9 concentration in the supernatant was determined by ELISA. ( d ) IL-17- and IL-9-producing cells were analysed by FACS. Numbers in quadrants indicate percentage of cells and are summarized in e . ( f ) CD4 + T cells were cultured under Th17/Th9 conditions (αCD3+IL-4, TGFβ, IL-6, IL-1β, IL-23 and anti-IFNγ)±NO. Percentage of cells producing IL-9 and IL-17 was determined by FACS. ( g ) IL-9 and IL-17 concentrations in the culture supernatant was assayed by ELISA. Data are representative of at least three independent experiments; Mean±s.e.m., n =3; * P <0.05, ** P <0.01, *** P <0.001 using a two-way analysis of variance ( b , c , e ) or a two-tailed unpaired Student’s t -test ( g ). Hprt, hypoxanthine-guanine phosphoribosyltransferase. Full size image Characterization of NO-induced Th9 cells We next investigated the role of NO on Th9 cell differentiation under Th9 polarizing culture conditions. CD4 + T cells were purified from naive BALB/c or B6 mice and cultured for up to 6 days with anti-CD3/CD28 antibodies+TGFβ, IL-4 and graded concentrations of NOC-18. NO enhanced T-cell proliferation as determined by carboxyfluorescein succinimidyl ester (CFSE) dilution ( Fig. 2a ). NO also markedly increased the percentage of IL-9 + T cells in a dose-dependent manner ( Fig. 2b ). The NO-induced enhancement of Th9 development was also evident in Il9 mRNA expression ( Fig. 2c ) and IL-9 protein produced in the culture supernatant ( Fig. 2d ). The expression PU.1 ( Sfpi1 ), a transcription factor, which has been reported to be required for Th9 development [4] , was also significantly increased by NO ( Fig. 2e ). Next we tested whether NO was able to enhance the expansion of the number of established Th9 cells. CD4 + T cells were polarized to Th9 by two rounds of culture, rested for 24 h and then re-cultured with anti-CD3/CD28 in the presence of graded concentrations of NOC-18. NO significantly enhanced the percentage of the polarized Th9 cells ( Fig. 2f ). Next, we examined whether NO can promote Th9 cell polarization in an antigen-specific manner. CD4 + T cells were purified from the spleen and lymph nodes (LN) of ovalbumin (OVA)-T cell receptor (TCR) transgenic mice (DO11.10) and cultured in vitro with OVA peptide and mitomycin C-treated APC in the presence of NOC-18. NO markedly increased the percentage of IL-9 + T cells ( Fig. 2g ) and IL-9 in the culture supernatant ( Fig. 2h ). We also tested the effect of NO on human Th9 cells. CD4 + T cells were purified from the peripheral blood of seven healthy volunteer donors and cultured with anti-human (h)CD3/hCD28 antibodies, hTGFβ and hIL-4 in the presence of NOC-18. NO significantly increased the percentage of IL-9 + T cells ( Fig. 2i,j ) and IL-9 in the culture supernatant ( Fig. 2k ). These results therefore demonstrate that NO potently enhances the development of murine and human Th9 cells in vitro at antigen-specific and polyclonal levels. 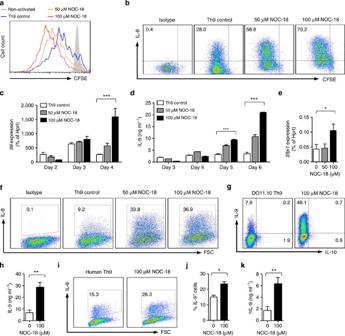Figure 2: NO enhances cell proliferation and IL-9 production during Th9 polarization. CFSE-labelled BALB/c CD4+T cells were cultured under Th9 polarizing conditions (flat-bottom 96-well plate with αCD3 and αCD28+IL-4, TGFβ)±NO. (a) T-cell proliferation (CFSE dilution) and (b) IL-9-producing cells were analysed by FACS on day 4. (c)Il9mRNA expression was determined by qPCR. (d) IL-9 concentrations in culture supernatant were assessed by ELISA. (e)Sfpi1mRNA was determined by qPCR on day 2. Similar results were obtained with cells from C57BL/6 mice. (f) Effect of NO on polarized Th9 cells. CD4+T cells were polarized 2 × as above, washed and re-cultured±NO for a further 4 days. Percentage of IL-9+cells was determined by FACS. (g,h) Effect of NO on antigen-specific Th9 cells. CD4+T cells purified from DO11.10 mice were cultured for two rounds under Th9 polarization conditions with APC and 1 μM of OVA323-339peptide±NO. IL-9- and IL-10-producing cells were analysed by FACS on day 2 of the second round (g), and IL-9 concentration in the supernatant was assessed by ELISA (h). CD4+T cells purified from total human peripheral blood mononuclear cells (PBMC) (n=7) were cultured with autologous APC, αhCD3, αhCD28+ hIL-4 and hTGF-β±NO. (i,j) Percentage of IL-9+cells analysed by FACS on day 4, and (k) IL-9 concentrations in supernatants determined by ELISA on day 5. Data are representative of three independent experiments (mouse cells); mean±s.e.m.,n=3, *P<0.05, **P<0.01, ***P<0.001 using a two-way analysis of variance (c,d,e) or a two-tailed unpaired Student’st-test (h,j,k). Figure 2: NO enhances cell proliferation and IL-9 production during Th9 polarization. CFSE-labelled BALB/c CD4 + T cells were cultured under Th9 polarizing conditions (flat-bottom 96-well plate with αCD3 and αCD28+IL-4, TGFβ)±NO. ( a ) T-cell proliferation (CFSE dilution) and ( b ) IL-9-producing cells were analysed by FACS on day 4. ( c ) Il9 mRNA expression was determined by qPCR. ( d ) IL-9 concentrations in culture supernatant were assessed by ELISA. ( e ) Sfpi1 mRNA was determined by qPCR on day 2. Similar results were obtained with cells from C57BL/6 mice. ( f ) Effect of NO on polarized Th9 cells. CD4 + T cells were polarized 2 × as above, washed and re-cultured±NO for a further 4 days. Percentage of IL-9 + cells was determined by FACS. ( g , h ) Effect of NO on antigen-specific Th9 cells. CD4 + T cells purified from DO11.10 mice were cultured for two rounds under Th9 polarization conditions with APC and 1 μM of OVA 323-339 peptide±NO. IL-9- and IL-10-producing cells were analysed by FACS on day 2 of the second round ( g ), and IL-9 concentration in the supernatant was assessed by ELISA ( h ). CD4 + T cells purified from total human peripheral blood mononuclear cells (PBMC) ( n =7) were cultured with autologous APC, αhCD3, αhCD28+ hIL-4 and hTGF-β±NO. ( i , j ) Percentage of IL-9 + cells analysed by FACS on day 4, and ( k ) IL-9 concentrations in supernatants determined by ELISA on day 5. Data are representative of three independent experiments (mouse cells); mean±s.e.m., n =3, * P <0.05, ** P <0.01, *** P <0.001 using a two-way analysis of variance ( c , d , e ) or a two-tailed unpaired Student’s t -test ( h , j , k ). Full size image NO-induced Th9 cell differentiation is IL-2 dependent We next investigated the mechanism by which NO enhances Th9 differentiation. Since IL-2 has been shown to increase Th9 development [13] and we have confirmed this in our own culture conditions ( Supplementary Fig. 2 ), we first examined the role of IL-2 in NO-induced Th9 development. CD4 + T cells were polarized under Th9 conditions in the presence of graded concentrations of NOC-18. The cells were cultured up to 6 days and the IL-2 expression was analysed. Il2 mRNA was clearly increased by the presence of NO ( Fig. 3a ). The percent of IL-2 + , IL-9 + and IL-2/IL-9 double-positive T cells were also markedly increased ( Fig. 3b ), together with the concentrations of IL-2 in the culture supernatant ( Fig. 3c ). Importantly, the enhancement of Th9 differentiation by NO was completely blocked by the presence of a neutralizing anti-IL-2 antibody ( Fig. 3d ). These results therefore demonstrate that the enhancement of Th9 differentiation by NO is IL-2 dependent and not via an additional pathway. CD25 expression was not affected by NO; all cells were 99% CD25 + after culture with or without NOC-18. 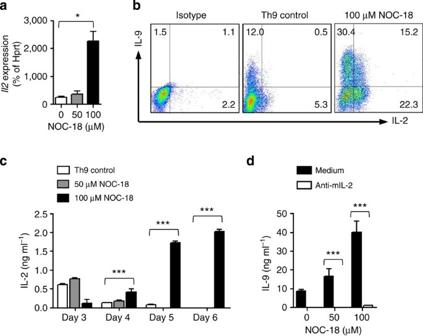Figure 3: Upregulation of Th9 cell polarization by NO is IL-2 dependent. C57BL6 CD4+T cells were cultured under Th9 polarizing conditions±NO. (a)Il2mRNA was determined by qPCR on day 2. (b) IL-9- and IL-2-producing cells were analysed by FACS on day 4. (c) IL-2 in cell culture supernatants was determined by ELISA. (d) IL-9 concentrations in the supernatant of Th9-polarized cells cultured in the presence of αIL-2 antibodies (20 μg ml−1) were determined on day 5. Data are representative of at least three independent experiments; mean±s.e.m., *P<0.05, ***P<0.001 using a two-way analysis of variance. Figure 3: Upregulation of Th9 cell polarization by NO is IL-2 dependent. C57BL6 CD4 + T cells were cultured under Th9 polarizing conditions±NO. ( a ) Il2 mRNA was determined by qPCR on day 2. ( b ) IL-9- and IL-2-producing cells were analysed by FACS on day 4. ( c ) IL-2 in cell culture supernatants was determined by ELISA. ( d ) IL-9 concentrations in the supernatant of Th9-polarized cells cultured in the presence of αIL-2 antibodies (20 μg ml −1 ) were determined on day 5. Data are representative of at least three independent experiments; mean±s.e.m., * P <0.05, *** P <0.001 using a two-way analysis of variance. Full size image NO-induced Th9 development is STAT5- and IRF4 dependent IL-2 activates the phosphorylation of STAT5 (refs 22 , 23 , 24 , 25 , 26 ), which has recently been shown to be important for IL-9 synthesis [27] . We therefore reasoned that pSTAT5 might be important in NO-induced Th9 differentiation. CD4 + T cells were cultured under Th9 polarizing conditions with NOC-18, and the percentage of pSTAT5 + cells was analysed by FACS. NO clearly increased the percentage of pSTAT5 + T cells in IL-9 + as well as IL-9 − cell populations ( Fig. 4a ). To directly determine the role of STAT5 in NO-induced Th9 differentiation, we cultured purified CD4 + T cells from Stat5 −/− mice under Th9 polarizing conditions in the presence of NOC-18. The percentage of IL-9 + cells was significantly reduced in Stat5 −/− cells compared with wild-type (WT) cells ( Fig. 4b ). Interestingly, STAT5-deficient T cells also exhibited significantly less IL-2 + T cells when cultured under these conditions ( Fig. 4c ), indicating that STAT5 functions as an amplifier for the auto-induction loop of IL-2. 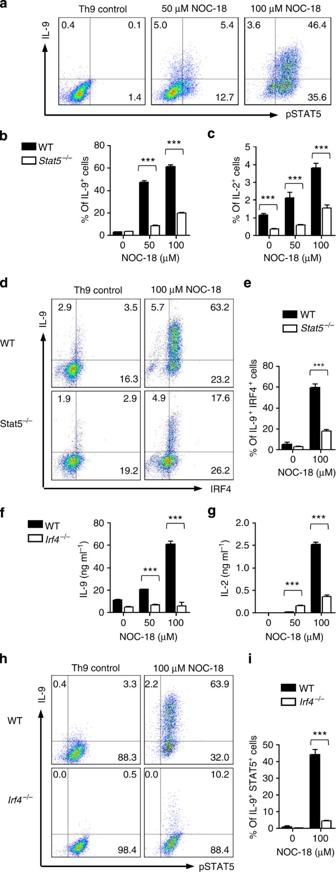Figure 4: Upregulation of Th9 polarization by NO depends on IRF4 and STAT5. CD4+T cells from WT,Stat5−/−orIrf4−/−mice were cultured under Th9 polarizing conditions with graded concentration of NO. (a) IL-9+and pSTAT5+cells were analysed by FACS on day 4. (b,c) Percentage of IL-9+and IL-2+T cells from WT andStat5−/−mice polarized under Th9 conditions with NO analysed by FACS on day 4. (d,e) Percentage of IL-9+IRF4+T cells from WT andStat5−/−mice cultured±NO for 4 days under Th9 conditions analysed by FACS. (f,g) Concentrations of IL-9 and IL-2 in the supernatants of T cells from WT andIrf4−/−mice cultured under Th9 conditions were determined by ELISA. (h,i) Percentage of IL9+pSTAT5+T cells from WT andIrf4−/−mice cultured under Th9 conditions was analysed by FACS. Data are representative or pool of at least three independent experiments; mean±s.e.m., ***P<0.001 using a two-way analysis of variance. Figure 4: Upregulation of Th9 polarization by NO depends on IRF4 and STAT5. CD4 + T cells from WT, Stat5 −/− or Irf4 −/− mice were cultured under Th9 polarizing conditions with graded concentration of NO. ( a ) IL-9 + and pSTAT5 + cells were analysed by FACS on day 4. ( b , c ) Percentage of IL-9 + and IL-2 + T cells from WT and Stat5 −/− mice polarized under Th9 conditions with NO analysed by FACS on day 4. ( d , e ) Percentage of IL-9 + IRF4 + T cells from WT and Stat5 −/− mice cultured±NO for 4 days under Th9 conditions analysed by FACS. ( f , g ) Concentrations of IL-9 and IL-2 in the supernatants of T cells from WT and Irf4 −/− mice cultured under Th9 conditions were determined by ELISA. ( h , i ) Percentage of IL9 + pSTAT5 + T cells from WT and Irf4 −/− mice cultured under Th9 conditions was analysed by FACS. Data are representative or pool of at least three independent experiments; mean±s.e.m., *** P <0.001 using a two-way analysis of variance. Full size image We also investigated the role of IRF4, a key downstream molecule of STAT5 (ref. 27 ) and an important transcription factor for the induction of IL-9 (ref. 5 ). CD4 + T cells from WT or Stat5 −/− mice were cultured under Th9 polarizing conditions in the presence of NOC-18, and the level of intracellular IRF4 expression was analysed by FACS. NO markedly increased the differentiation of IRF4 + T cells in the WT cell population but only modestly in STAT5-deficient cells ( Fig. 4d ). Furthermore, NO strongly increased the frequency of IL-9/IRF4 double-positive T cells in the WT cells but only marginally in the STAT5-deficient cells ( Fig. 4e ). To directly determine the role of IRF4 in NO-induced Th9 cell differentiation, we cultured CD4 + T cells from Irf4 −/− mice under Th9 polarizing conditions in the presence of NOC-18. CD4 + T cells from Irf4 −/− mice produced significantly less IL-9 compared with cells from the WT mice ( Fig. 4f ). Furthermore, Irf4 −/− T cells also produced markedly reduced levels of IL-2 ( Fig. 4g ), indicating that IRF4 is also a mediator of the IL-2 self-amplification loop. The Irf4 −/− cells also developed less percentage of IL-9 + /pSTAT5 + T cells ( Fig. 4h,i ). However, the frequency of total pSTAT5 + T cells (IL-9 +/− ) was the same in the WT or Irf4 −/− T cells when cultured with NO under Th9 polarizing conditions ( Fig. 4h ), confirming that IRF4 functions downstream of STAT5 in the induction of IL-9. Together, these results demonstrate that NO-induced Th9 differentiation is also dependent on the activation of STAT5 and IRF4. NO-induced Th9 differentiation is p53 dependent Results obtained above so far indicate that NO induces IL-2 synthesis, which then activates STAT5 phosphorylation leading to the induction of IRF4 that promotes IL-9 synthesis. We then investigated the mechanism by which NO induces IL-2 synthesis. In a previous study, we reported that low doses of NO could activate IL-12Rβ expression via cyclic guanosine monophosphate (cGMP) [28] . We therefore examined the role of cGMP in the present culture system. We found that 8-bromo-GMP, at concentrations (3–5 mM) known to activate several downstream events of cGMP, was not able to enhance Th9 differentiation or IL-2 synthesis ( Supplementary Fig. 3a,b ). Furthermore, ODQ (1-H-oxdiazolo-[1,2,4]-[4,3-α]quinoxalin-1-one, 5–10 μM) a potent inhibitor of cyclic guanylate cyclase, the enzyme catalyzing cGMP synthesis, also had no effect on NO-mediated enhancement of Th9 differentiation or IL-2 production ( Supplementary Fig. 3c,d ). Thus, the effect of NO on Th9 differentiation is unlikely to be mediated by the induction of cGMP. In another previous report [29] , we demonstrated that NO induced a population of Foxp3-negative Tregs (NO-Tregs) via the activation of p53 , the tumour suppressor gene, that increased IL-2 synthesis. We therefore investigated the possibility that p53 may also have a role in the NO-mediated enhancement of Th9 differentiation. Naive C57BL/6 CD4 + T cells were cultured under Th9 polarizing conditions in the presence of NOC-18, and the expression of p53 was analysed by FACS. NO induced substantial expression of p53 ( Fig. 5a ). To directly test the role of p53 in our culture system, CD4 + T cells from p53 −/− or littermate WT mice were cultured under Th9 polarizing conditions in the presence of NOC-18. CD4 + T cells from p53 −/− mice produced significantly less IL-9 ( Fig. 5b ) and IL-2 ( Fig. 5c ) compared with that of the WT mice. It should be noted that p53 −/− cells retained a low capacity to polarize to Th9 cells, indicating that a p53-independent pathway may also be involved in NO-mediated enhanced Th9 polarization. The p53-deficient CD4 + T cells also generated significantly less IL-9 + as well as IL-9 + pSTAT5 + double-positive T cells compared with that of the WT mice ( Fig. 5d,e ). The frequency of total pSTAT5 + cells, however, remained unchanged, suggesting that the effect of p53 on pSTAT5 is confined to Th9 cells in our system. We then investigated whether recombinant IL-2 can reverse the reduced ability of p53 −/− cells to generate IL-9 with or without NO. As expected, NO induced a low frequency of Th9 cells from CD4 + T cells of p53 −/− mice. This was markedly increased by the addition of recombinant murine IL-2 in the culture in the absence of NO. This increase was even more evident in the presence of NO ( Fig. 5f,g ). NO induced lower levels of IRF4 in p53 −/− cells compared with WT cells ( Fig. 5h ). However, exogenous murine IL-2 was also able to reverse the reduced ability of NO to enhance IRF4 expression ( Fig. 5h ). These results therefore indicate that p53 is a key molecule for the NO-mediated enhancement of Th9 differentiation, and p53 is likely upstream of the cascade of events leading to the enhanced Th9 development. 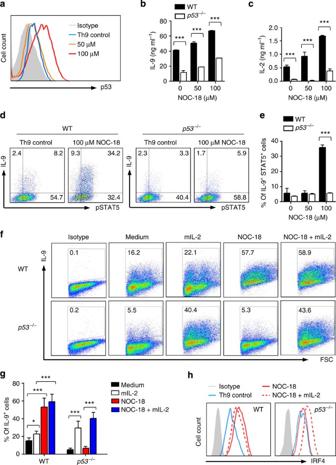Figure 5: NO-induced up-regulation of Th9 polarization is p53-dependent. CD4+T cells from WT andp53−/−B6 mice were cultured under Th9 polarizing conditions±NO. (a) The expression of p53 in WT Th9 cells on day 4 was analysed by FACS. Concentrations of IL-9 (b) and IL-2 (c) in the culture supernatants of WT andp53−/−cells on day 5 were determined by ELISA. (d,e) Percent of IL-9+and pSTAT5+T cells from WT andp53−/−mice polarized under Th9 conditions was analysed by FACS on day 4. Representative (f) and percent (g) of IL-9+T cells from WT orp53−/−mice cultured under Th9 conditions in the presence of NO with or without IL-2 are shown. mIL-2, murine IL-2. (h) Expression of IRF4 in the Th9 cells from WT andp53−/−mice polarized under Th9 conditions±NO±IL-2 was analysed by FACS. Data are representative or pool of at least three experiments, mean±s.e.m.,n=3, *P<0.05, ***P<0.001 using a two-way analysis of variance. Figure 5: NO-induced up-regulation of Th9 polarization is p53-dependent. CD4 + T cells from WT and p53 −/− B6 mice were cultured under Th9 polarizing conditions±NO. ( a ) The expression of p53 in WT Th9 cells on day 4 was analysed by FACS. Concentrations of IL-9 ( b ) and IL-2 ( c ) in the culture supernatants of WT and p53 −/− cells on day 5 were determined by ELISA. ( d , e ) Percent of IL-9 + and pSTAT5 + T cells from WT and p53 −/− mice polarized under Th9 conditions was analysed by FACS on day 4. Representative ( f ) and percent ( g ) of IL-9 + T cells from WT or p53 −/− mice cultured under Th9 conditions in the presence of NO with or without IL-2 are shown. mIL-2, murine IL-2. ( h ) Expression of IRF4 in the Th9 cells from WT and p53 −/− mice polarized under Th9 conditions±NO±IL-2 was analysed by FACS. Data are representative or pool of at least three experiments, mean±s.e.m., n =3, * P <0.05, *** P <0.001 using a two-way analysis of variance. Full size image NO enhances p53 expression by nitrosylation of Mdm2 We next investigated the mechanism by which NO enhances the activity of p53. A key feature of the p53 response is p53 stabilization, leading to an increase in p53 steady-state levels [30] , [31] . In non-stressed cells, the level of p53 is controlled by the mouse double-minute 2 homologue (Mdm2). Mdm2, also known as E3 ubiquitin–protein ligase, is a highly conserved protein that in humans is encoded by the HDM2 gene. Mdm2 is an important negative regulator of p53 and functions both as an E3 ubiquitin ligase that recognizes the N-terminal transactivation domain of p53 and an inhibitor of p53 transcriptional activation [32] , [33] , [34] . Hdm2 can also regulate p53 by binding to p53 and inhibiting its transcriptional activity [35] . It has been demonstrated that NO nitrosylates a critical cysteine residue (C77) of Hdm2 and disrupts Hdm2-p53 binding. We therefore tested the possibility that NO enhances p53 expression by nitrosylation of Mdm2. C57BL/6 CD4 + T cells were polarized under Th9 polarizing conditions in the presence of NOC-18 and the cell lysate assayed for Mdm2-p53 binding by ELISA at various time points. NO markedly reduced Mdm2-p53 binding, evident at 6 h and sustained for at least 48 h ( Fig. 6a ). To ascertain that NO enhances Th9 differentiation via S-nitrosylation of Mdm2, we added excess amounts of cysteine into Th9 polarization culture. Exogenous cysteine significantly abrogated the NO-mediated inhibition of Mdm2-p53 binding ( Fig. 6b ; P <0.001). Cysteine also blocked the increase in the frequency of IL-9 + p53 + T cells induced by NO ( Fig. 6c ). To confirm these results, we chemically reversed the S-nitrosylation with ascorbate. This mild reductant abrogates the nitrosylation of thiols without affecting the ability to form disulphide bonds [36] . Ascorbate reversed NO-mediated inhibition of Mdm2-p53 binding ( Fig. 6b ) and limited the enhancement of the polarization of IL-9 + p53 + T cells ( Fig. 6c ). Furthermore, cysteine and ascorbate also inhibited the increase of the frequency of IL-9 + IL-2 + ( Fig. 6d ), IL9 + pSTAT5 + ( Fig. 6e ) and IL-9 + IRF4 + T cells ( Fig. 6f ). Together, these results demonstrate that NO enhances p53 expression by nitrosylation of cysteine of Mdm2 and blocking Mdm2-p53 binding. Interestingly, NO also enhanced STAT6 phosphorylation ( Supplementary Fig. 4a ), which was also reversed by cysteine and ascorbate ( Supplementary Fig. 4a,b ). 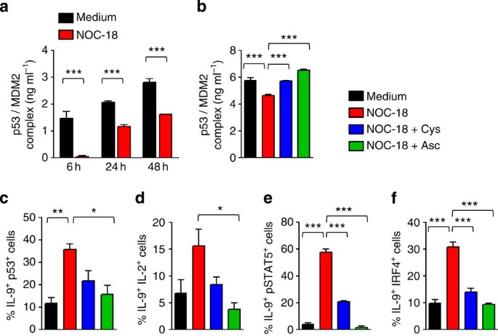Figure 6: NO enhances Th9 polarization via nitrosylation of MDM2-p53 complex. (a) BALB/c CD4+T cells were polarized under Th9 conditions±100 μM NOC-18. p53/MDM2 complex in the cell extracts were determined by ELISA. (b) CD4+T cells were polarized as above in the presence of cysteine (1 mM) or ascorbate (300 μM) for 24 h and the cell extracts analysed for p53/MDM2 complex. Percentage of IL-9+p53+T cells on day 4 (c), IL-9+IL-2+T cells on day 4 (d), IL-9+pSTAT5+T cells on day 5 (e), and IL-9+IRF4+T cells (f) on day 4 analysed by FACS. Data are representative or pooled of at least three experiments; mean±s.e.m.,n=3–5, *P<0.05, **P<0.01, ***P<0.001 using a two-way analysis of variance. Figure 6: NO enhances Th9 polarization via nitrosylation of MDM2-p53 complex. ( a ) BALB/c CD4 + T cells were polarized under Th9 conditions±100 μM NOC-18. p53/MDM2 complex in the cell extracts were determined by ELISA. ( b ) CD4 + T cells were polarized as above in the presence of cysteine (1 mM) or ascorbate (300 μM) for 24 h and the cell extracts analysed for p53/MDM2 complex. Percentage of IL-9 + p53 + T cells on day 4 ( c ), IL-9 + IL-2 + T cells on day 4 ( d ), IL-9 + pSTAT5 + T cells on day 5 ( e ), and IL-9 + IRF4 + T cells ( f ) on day 4 analysed by FACS. Data are representative or pooled of at least three experiments; mean±s.e.m., n =3–5, * P <0.05, ** P <0.01, *** P <0.001 using a two-way analysis of variance. Full size image NO enhances the expression of TGFβR and IL-4R TGFβ and IL-4 are essential for the polarization of Th9 cells [2] , [3] , [13] . Moreover, STAT6 phosphorylation is a key downstream event of IL-4 signalling [37] , [38] , [39] . We therefore investigated whether NO also has an effect on the expression of TGFβR and IL-4Rα on CD4 + T cells during Th9 polarization. Purified CD4 + T cells were cultured under Th9 conditions with or without NOC-18. NO markedly increased the percentage of Th9 cells expressing TGFβR2 ( Supplementary Fig. 5a ). It should be noted that not all Th9 + cells expressed TGFβR2. This may reflect the dynamic nature of this receptor, being internalized and re-expressed continuously [40] . The increase of Tgfβr2 and Il4r α mRNA expression was also evident ( Supplementary Fig. 5b ). These results therefore demonstrate that the direct enhancement of TGFβR and IL-4Rα expression may be an additional pathway by which NO promotes the differentiation of Th9 cells. This observation may explain the low but significant level of enhanced Th9 differentiation in response to NO in the p53 −/− cells ( Fig. 4b ) above. The role of NO on Th9 cells function in vivo Next, we investigated the in vivo relevance of our observation. Th9 cells have an important role in allergic diseases, including airway inflammation [4] , [5] , [12] . We therefore examined the effect of NO in an experimental model of allergic airway inflammation using the OVA priming and challenge system. C57BL/6 mice were immunized intraperitoneally (i.p.) with OVA plus Alum and challenged intranasally (i.n.) with OVA on days 7, 10, 13, 16 and 19. The mice were also injected subcutaneously (s.c.) every other day with NOC-18 (10 mg kg −1 ) or phosphate-buffered saline (PBS). Mice were killed on day 20 and the bronchoalveolar lavage (BAL) was collected for analysis. Mice treated with NOC-18 showed significantly increased eosinophilia in the BAL compared with PBS-treated control mice ( Fig. 7a ). The BAL fluid from NOC-18-treated mice also contained significantly more IL-9 compared with that of the PBS-treated control mice ( Fig. 7b ). IL-13 was also detected in the BAL of the OVA-immunized and challenged mice but the level of IL-13 was not affected by NOC-18 treatment, indicating that NO has little effect on IL-13 synthesis. 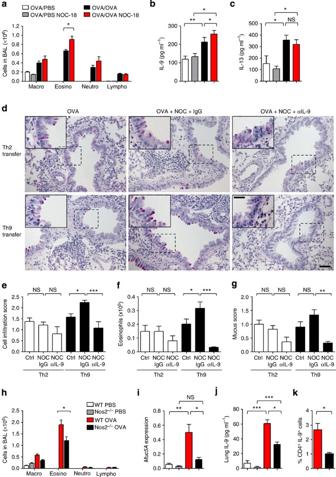Figure 7: NO enhances IL-9 production and Th9 frequency and exacerbates allergic airway inflammation in mice. (a–c) OVA-immunized C57BL/6 mice were challenged with OVA and injected s.c. every 2 days with NOC-18. Differential cell counts (a), IL-9 concentration (b) and IL-13 content (c) in the BAL fluid were determined 24 h after the last challenge. (d–g) CD4+T cells from OT-II mice were polarized to Th9 or Th2 cells and adoptively transferred i.n. to naive recipient mice that were then challenged i.n. with OVA±NOC-18. Some mice were injected i.p. with αIL-9 antibody or IgG. Periodic acid Schiff reagent (PAS) staining were performed on lung sections obtained 24 h after the last challenge (d). Scale bars represent 100 and 400 μm for the insert. Cell infiltration in the lungs (e), Eosinophils in BAL fluids (f), and mucus score in the lung tissues (g) were measured. (h–k) WT andNos2−/−mice were immunized s.c. with OVA and challenged i.n. with OVA or PBS. BAL was analysed by differential cell count (h). Lungs were analysed forMucin5AmRNA expression by qPCR (i) and IL-9 concentration by ELISA (j). Percentage of Th9 (CD4+/IL9+) cells in the draining lymph node was analysed by FACS (k). Experiments were performed at least twice; data are mean±s.e.m.,n=5–6 mice per group; *P<0.05, **P<0.01, ***P<0.001 using two-way analysis of variance. NS, not significant. Figure 7: NO enhances IL-9 production and Th9 frequency and exacerbates allergic airway inflammation in mice. ( a – c ) OVA-immunized C57BL/6 mice were challenged with OVA and injected s.c. every 2 days with NOC-18. Differential cell counts ( a ), IL-9 concentration ( b ) and IL-13 content ( c ) in the BAL fluid were determined 24 h after the last challenge. ( d – g ) CD4 + T cells from OT-II mice were polarized to Th9 or Th2 cells and adoptively transferred i.n. to naive recipient mice that were then challenged i.n. with OVA±NOC-18. Some mice were injected i.p. with αIL-9 antibody or IgG. Periodic acid Schiff reagent (PAS) staining were performed on lung sections obtained 24 h after the last challenge ( d ). Scale bars represent 100 and 400 μm for the insert. Cell infiltration in the lungs ( e ), Eosinophils in BAL fluids ( f ), and mucus score in the lung tissues ( g ) were measured. ( h – k ) WT and Nos2 −/− mice were immunized s.c. with OVA and challenged i.n. with OVA or PBS. BAL was analysed by differential cell count ( h ). Lungs were analysed for Mucin5A mRNA expression by qPCR ( i ) and IL-9 concentration by ELISA ( j ). Percentage of Th9 (CD4 + /IL9 + ) cells in the draining lymph node was analysed by FACS ( k ). Experiments were performed at least twice; data are mean±s.e.m., n =5–6 mice per group; * P <0.05, ** P <0.01, *** P <0.001 using two-way analysis of variance. NS, not significant. Full size image To confirm the role of NO in Th9 function in this model, we polarized OVA-specific OT-II transgenic CD4 + T cells to Th9 cells in vitro . The polarized cells were >95% IRF4 + and were negative for IL-13, IL-10, IL-4, IFNγ, IL-17, Foxp3, T-bet or RORγt. As control, we also polarized OT-II cells to Th2 cells as described previously [41] . The cells were adoptively transferred i.n. to naive C57BL/6 mice, which were then challenged i.n. with OVA and treated i.n. with NOC-18 or PBS. Some mice were also injected i.p. with anti-IL-9 antibody or control IgG. OVA-challenged mice that had received Th9 cells developed symptoms of airway inflammation, including increased inflammatory cell infiltration in the lungs ( Fig. 7d , periodic acid Schiff reagent staining, and Fig. 7e ), the number of eosinophils in BAL ( Fig. 7f ) and mucus production in the lungs ( Fig. 7g ), which were all exacerbated by NO treatment. Th2 cells also induced eosinophilia, inflammatory cells infiltration and mucus production in the lungs. However, these parameters were not affected by the NOC-18 treatment ( Fig. 7d–g ). Treatment of recipient mice with a neutralizing anti-IL-9 antibody strongly ameliorated eosinophilia, lung inflammation and mucus production induced by Th9 cells, but this antibody had a only minor effect on the Th2-induced airway inflammation ( Fig. 7d–g ). To demonstrate an endogenous role of NO in this model, we immunized and challenged Nos2 −/− or WT mice with OVA. Nos2 −/− mice showed significantly less eosinophilia in the BAL ( Fig. 7h ) and Mucin5A expression in the lungs ( Fig. 7i ) compared with that of the WT mice. The attenuated airway inflammation in the Nos2 −/− mice was accompanied by a significant reduction in the level of IL-9 in the lungs of Nos2 −/− mice compared with the WT mice ( Fig. 7j ). Importantly, OVA-immunized Nos2 −/− mice also produced significantly less CD4 + IL-9 + T cells in the draining lymph nodes compared with WT mice ( Fig. 7k and Supplementary Fig. 6a ). There was, however, no difference in the level of Nos3 expression between the OVA-immunized and challenged Nos2 −/− and WT mice ( Supplementary Fig. 6b ), showing that Nos2 -deficiency did not lead to an elevated Nos3 expression. CD4 + T cells from Nos2 −/− and WT mice produced similar percentage of Th9 cells and secreted equivalent amounts of IL-9 when polarized under Th9 conditions in vitro ( Supplementary Fig. 6c,d ). These results are consistent with the relatively low level of NO production by T cells, and the notion that in vivo NO is likely provided by other cell types including endothelial and myeloid cells. Together, these result demonstrate that NO has an important endogenous role in the induction of airway inflammation, and that this effect is associated with the enhanced Th9 polarization in vivo . Data presented in this report demonstrate a hitherto unrecognized role of NO in the induction of Th9 cells. This finding expands the regulatory role of NO in the immune system, linking NO to the differentiation and function of the latest subset of T helper cells and the endogenous effect of NO in airway inflammation. We also provide the molecular mechanism by which NO potentiates the expansion and maintenance of Th9 ( Fig. 8 ). NO nitrosylates cysteine residues of Mdm2, a repressor of p53, thereby reduces the binding of Mdm2 to p53, and thus stabilizes and increases the level of p53, leading to the increased production of IL-2. IL-2, via its receptor CD25, induces the phosphorylation of STAT5, which increases the expression of IRF4 that can enhance IL-9 synthesis by binding to the promoter of Il9 . pSTAT5 may also bind directly to the promoter of Il9 and enhance IL-9 synthesis [42] . 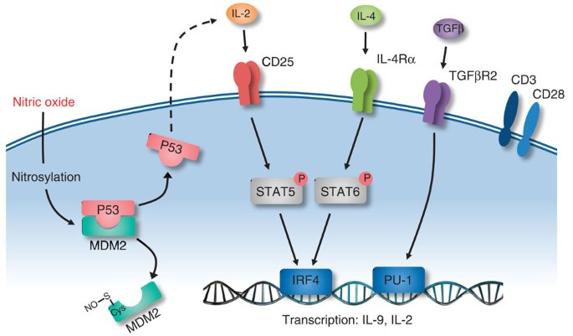Figure 8: Schematic representation of the mechanism of NO-mediated enhancement of Th9 polarization. NO nitrosylates cysteine of MDM2 leading to the release of p53 from the MDM2-p53 complex. p53 induces IL-2 synthesis that binds to CD25 (IL-2R α-chain) leading to STAT5 phosphorylation that activates IRF4, which binds to the promoter ofIl9for enhanced IL-9 transcription. NO also promotes IL-4Rα expression, thus stimulates STAT6 phosphorylation that can also induce IRF4 expression. NO can also enhance TGFβR2 expression leading to the activation of PU.1 that can promote IL-9 transcription by binding toIl9promoter. NO-mediated Th9 promotion is dependent on conventional TCR and CD28 activation. Figure 8: Schematic representation of the mechanism of NO-mediated enhancement of Th9 polarization. NO nitrosylates cysteine of MDM2 leading to the release of p53 from the MDM2-p53 complex. p53 induces IL-2 synthesis that binds to CD25 (IL-2R α-chain) leading to STAT5 phosphorylation that activates IRF4, which binds to the promoter of Il9 for enhanced IL-9 transcription. NO also promotes IL-4Rα expression, thus stimulates STAT6 phosphorylation that can also induce IRF4 expression. NO can also enhance TGFβR2 expression leading to the activation of PU.1 that can promote IL-9 transcription by binding to Il9 promoter. NO-mediated Th9 promotion is dependent on conventional TCR and CD28 activation. Full size image Although we have focused on the NO→Mdm2→p53→IL-2-STAT5→IRF4→Th9 axis, other contributing signalling pathways are not excluded. For example, we have shown that NO enhances the expression of TGFβR and Il4r α, Sfpi1 (PU.1) and pSTAT6 in Th9 cells. It is thus likely that PU.1 activated by TGFβ could contribute to the promotion of IL-9 synthesis [43] . Furthermore, the increased IL-4Rα expression could lead to the phosphorylation of STAT6 that enhances IL-9 synthesis by binding directly to the promoter of Il9 (ref. 42 ) or indirectly via IRF4 (refs 42 , 43 ). IL-2 has also been reported to activate STAT6 (ref. 44 ). OX40 signalling has recently been reported to favour the induction of Th9 and airway inflammation [45] . However, in our experimental system, we did not use APCs and thus precluded an effect on OX40. In a previous report [29] , we showed that NO inhibits Th17 induction by downregulating the aryl hydrocarbon receptor. We show here that NO can elevate the phosphorylation of STAT5 that has been shown to be an inhibitor of IL-17 synthesis [46] . Thus, the induction of pSTAT5 under the Th9 polarizing conditions could be an additional mechanism by which NO suppresses Th17 differentiation. In an acute (7 days) papain-induced lung inflammation model in mice, Wilhelm et al. [40] reported that IL-9 production was largely restricted to innate lymphoid cells. IL-9 production by innate lymphoid cells depended on IL-2 and was rapidly lost in favour of IL-13 and IL-5. In a murine model of allergic inflammation, Jones et al. [12] reported that Th9 cells were rapidly generated in vivo after exposure to house dust mite (HDM). Interestingly, Th9 cell recruitment to the lung peaked 1 week after initial allergen administration, before Th2 cell recruitment. In contrast, in a chronic allergen exposure mouse model using the clinically relevant antigen Aspergillus fumigatus to determine the kinetics of Th9 development in vivo , Kerzerho et al. [47] reported that Th9 began to appear in the lungs from day 39 and sustained at least till day 46. These IL-9-producing CD4 + T cells did not co-express IL-4, IL-13 or IL-10, a phenotype consistent with the murine and human Th9 cells we observed here. Our data show that NO enhances not only the differentiation of Th9 but also the maintenance of Th9 cells. Although NOS2 is not readily detected in human peripheral blood monocytes, the overall role of NOS2 in humans is not in doubt. NOC-18 at a concentration of 100–200 μM consistently releases 200–400 nM of NO with a half-life of 20 h (ref. 48 ). This dose of NO occurs in vivo in sites of infection and inflammation [49] , and has been used routinely in experiments in vitro [29] , [49] . The expression of NOS2 in the site of inflammation has also been extensively reported [50] , [51] . Bronchial biopsy specimens from human asthmatic patients show increased expression of Il9 and its receptor compared with healthy controls [11] , [52] , [53] , [54] . A humanized monoclonal anti-IL-9 antibody has recently been used in two phase II clinical trials in asthmatics with evidence of clinical activity [55] . In the present report, we demonstrate an endogenous enhancing role of NO in Th9 differentiation and airway inflammation. NO is detected in the exhaled air of animals and humans [56] . A marked increase in the concentration of exhaled NO has been reported in asthmatic patients [57] , [58] , and an association of NO with asthmatic inflammation has long been recognized [59] . Although not widely implemented, fraction of exhaled NO has emerged in recent years as a potential useful, rapid and noninvasive biomarker for assessing airway inflammation, particularly for patients who would be responsive to inhaled corticosteroid treatment [60] , [61] , [62] . The mechanism of NO causes severe asthma is hitherto unclear. This is counter-intuitive since NO itself is a bronchodilator [63] . Our data indicate that NO may act via promoting the differentiation of Th9 cells. This finding may, at least in part, explain the lack of effectiveness of anti-IL-5 monoclonal antibody (mepolizumab) in treating asthma. Mepolizumab significantly reduces blood and sputum eosinophils without affecting fraction of exhaled NO levels [64] . Data reported here therefore not only reveal a hitherto unrecognized mechanism of Th9 regulation by NO but also provide a long-sought explanation by which NO exacerbates airway inflammation. Mice BALB/c and C57BL/6 (B6) mice were obtained from Harlan, UK. Nos2 −/− mice, DO11.10 mice (BALB/c background) and OT-II mice (B6 background) were originally obtained from the Jackson Laboratory. Irf4 −/− mice (B6 background) were obtained as described previously [65] . Cells from the p53 −/− mice (B6 background) were provided by Dr Ewen McGregor (University of Glasgow). Cells from the Stat5 −/− mice (B6 background) were provided by Dr Arian Laurence (National Institutes of Health, Bethesda). Nos2 −/− mice (B6 background) were obtained from the Jackson Laboratory. Male and female mice were used at the age of 6–10 weeks. Cells from BALB/c and C57BL/6 mice gave similar results. All animal experiments were performed according to institutional guidelines in the Ribeirão Preto Medical School, University of São Paulo, Brazil (USP number 038/2009) and in accordance with the French ethical and animal experiments regulations in the project approved by the Ethics Committee for Animal Experimentation of CNRS Campus Orleans (N° CLE CCO 2012-050, UMR7355, Orleans, France). In vitro murine cell cultures CD4 + T cells were purified from the pool of spleens and lymph nodes of naive mice by negative selection (routine purity >98%) using an AutoMacs (Miltenyi Biotec). Culture medium was RPMI-1640 supplemented with 10% (vol/vol) faetal calf serum (FCS) (Lonza), 2 mM L -glutamine, 100 U ml −1 penicillin, 100 μg ml −1 streptomycin, and 0.05 M 2-mercaptoethanol. For Th17 cell differentiation, 5 × 10 5 cells ml −1 were cultured in round-bottom 96-well plates with mitomycin C-treated spleen cells (APCs, 1:1 ratio APC:T cells), 1 μg ml −1 soluble anti-CD3, 1 ng ml −1 TGFβ, 10 ng ml −1 IL-6, 10 ng ml −1 IL-1β, 10 μg ml −1 anti-IFNγ and 10 μg ml −1 anti-IL-4. For Th9 cell differentiation, 1 × 10 6 cells ml −1 were cultured for up to 6 days in flat-bottom 96-well plates with 3 μg ml −1 plate-bound anti-CD3, 1.5 μg ml −1 soluble anti-CD28, 5 ng ml −1 TGFβ, 10 ng ml −1 IL-4 and 10 μg ml −1 anti-IFNγ. In some experiments, CD4 + T cells were cultured under Th9/17 conditions in flat-bottom plate with plate-bound anti-CD3 (3 μg ml −1 ) and anti-CD28 (1.5 μg ml −1 ), 1 ng ml −1 TGFβ, 10 ng ml −1 IL-6, 10 ng ml −1 IL-1β, 10 ng ml −1 IL-4 and 10 μg ml −1 anti-IFNγ. NO donor (NOC-18) was added only once at the beginning of the culture (immediately before cells) at the indicated doses. In some experiments, IL-2 (5–20 ng ml −1 ), anti-IL-2 antibody (10 μg ml −1 ), cysteine (1 mM, Sigma) or ascorbate (100–300 μM, Sigma) was also added in the culture. Cultures were incubated at 37 °C in 5% CO 2 for up to 6 days. At the end of cultures, supernatants were collected for cytokine assay using ELISA, and the cells were used for RNA extraction or FACS analysis. Th9 cells polarized under the conditions indicated in the legend to Fig. 6 were harvested at 6–72 h. Cell lysates were prepared for Mdm2-p53 binding assay (Enzo Life Sciences) as per instructions of the manufacturer. Cell division was determined by labelling CD4 + T cells with CFSE (Molecular Probes, Inc.) by flow cytometry at the indicated time points. All cytokines and antibodies were obtained from PeproTech and R&D Systems. Human cell culture Peripheral blood was obtained from healthy donors ( n =7) with informed consent (WSBTS-12-10). Mononuclear cells were purified by Ficoll-Paque Plus (GE Healthcare), followed by CD4 + T-cell isolation using AutoMacs. The cells were cultured (1 × 10 6 ml −1 ) for 5 days in round-bottom 96-well plates (Costar) with mitomycin C-treated autologous APC (1 × 10 6 ml −1 ) together with soluble anti-hCD3 (1.5 μg ml −1 , Invitrogen) and anti-hCD28 (1 μg ml −1 , Invitrogen) plus hIL-4 (10 ng ml −1 , R&D Systems), hTGFβ (2.5 ng ml −1 , eBioscience), hIL-1β (10 ng ml −1 , R&D Systems), anti-hIFNγ (10 ng ml −1 , R&D Systems) in the presence of NOC-18. In some experiments, CD4 + T cells were cultured with anti-hCD3/CD28-conjugated Dynabeads (4 × 10 7 ml −1 , Invitrogen) instead of APC, with similar results. At the end of the culture, supernatants were harvested for ELISA and the cells were stained for intracellular cytokines. FACS analysis For measurement of intracellular cytokines, cells were stimulated for 4 h with phorbol 12-myristate 13-acetate (PMA) and ionomycin (both from Sigma) in the presence of GolgiStop (BD Biosciences). The cells were first stained for CD4, then permeabilized with Perm/Fix solution (eBioscience) and finally stained with antibodies against IL-17A, IL-9, IL-10, p53, pSTAT5, pSTAT6, IRF4 and TGFβR2 (eBioscience, Biolegend or R&D Systems). Isotype-matched rat anti-mouse antibodies (directly conjugated) were used as controls. Antibodies were routinely used in 1/100 dilution for 1 million cells. Data were acquired using a FACSCalibur (BD Biosciences) and analysed using FlowJo software (Tree Star). OVA-induced allergic airway inflammation Mice were sensitized i.p. on day 0 with 50 μg of OVA (grade V, Sigma-Aldrich) with 1.6 mg of alum adjuvant (Sigma-Aldrich). On days 7, 10, 13, 16 and 19, mice were challenged i.n. with 25 μg of OVA or PBS. In some experiments, NO donor (NOC-18, 10 mg kg −1 freshly diluted in PBS) was injected s.c. every 2 days. Control mice received the same volume of PBS. In some experiments, WT and Nos2 −/− mice were immunized s.c. with 10 μg of OVA in PBS on days 1 and 7, and challenged i.n. with 10 μg of OVA in PBS on day 14, 15 and 16. Mice were culled 24 h after the last challenge, and serum, BAL, lung and draining lymph nodes were collected for analysis. Th9 cell transfer CD4 + T cells purified from OT-II mice were cultured for 2 days with IL-4 (10 ng ml −1 ), TGFβ (5 ng ml −1 ), anti-IFNγ (20 μg ml −1 ), plate-bound anti-CD3 (3 μg ml −1 ) and soluble anti-CD28. Th9 cells were harvested, washed with PBS and 2 × 10 6 cells were adoptively transferred i.n. into naive C57BL/6 recipient mice. Mice were challenged i.n. with 10 μg of OVA on days 1, 2 and 3 after adoptive transfer. Simultaneously, mice received i.n. NOC-18 (10 mg kg −1 ) or PBS. In some experiments a neutralizing anti-IL-9 antibody (Clone 222622, R&D Systems) or a control antibody (rat IgG2b, R&D Systems) was given i.p. 30 min before each challenge. Animals were culled 24 h after the last challenge and the extent of airway inflammation was assessed in the BAL, lung and metiastinal lymph nodes (mLN). In some experiments, Th2 cells were also transferred and the recipients were treated similarly to those given Th9 cells. Th2 cells were generated as described previously [41] . In brief, CD4 + T cells were cultured for 2 days with plate-bound anti-CD3 and anti-CD28 plus IL-4, anti-IL-12 and anti-IFNγ. The cells were then harvested, washed and transferred [57] , [58] , [59] , [60] , [61] , [62] , [63] , [64] . BAL and lung analysis BAL fluid was obtained by four tracheal infusions of 0.5 ml PBS. After centrifugation for 10 min at 1,500 r.p.m., supernatant was stored at −20 °C for cytokine analysis and total cells were counted in Turks solution. Cytospin preparations were stained with Wright's stain (Diff-Quik, Dade Behring), and differential cell counts were obtained based on morphology and staining characteristics. For cytokine detection in total lung, the tissue was homogenized in 50 mM Tris·HCl, pH 7.5, 0.002% Tween 20 and protease inhibitor (Roche Applied Science). After centrifugation, supernatants were collected and stored at −80 °C. Lung histology Mice were perfused with 10 ml of PBS through the right ventricle. For histological analysis, a piece of lung was fixed overnight in 4% formaldehyde solution and embedded in paraffin. Lung sections (4 μm) were stained with haematoxylin and eosin or with periodic acid Schiff reagent. Histo-pathological assessment was performed blind on randomized sections. Inflammatory changes were graded using a semi-quantitative scale of 0–3 for perivascular and peri-bronchial cell infiltration and mucus production. Microarray analysis Total RNA was extracted using Qiagen RNeasy Mini kit (Qiagen), reverse-transcribed, followed by cDNA extraction with a PhaseLock gel (Eppendorf), and precipitated with ethanol and ammonium acetate. cRNA was transcribed with the MEGAscript high yield transcription kit (Ambion). The hybridization cocktail was prepared according to Affymetrix protocols (15 μg fragmented biotin-labelled cRNA spiked with Eukaryotic Hybridization control). The Murine Genome 430A version 2 GeneChip arrays (Affymetrix) were hybridized at 45 °C for 16 h, stained with streptavidin–phycoerythrin using the Affymetrix GeneChip Fluidics Workstation 400 and scanned on an Affymetrix GeneChip Scanner 3,000 (MG430Av2 arrays). Data were analysed using the Microarray Suite 5.0 software (Affymetrix) and deposited under the accession code E-MEXP-3959. Microarrays were globally normalized and scaled to a trimmed mean expression value of 200. Fold induction of individual gene between untreated and NO-treated Th17 cells was represented by the ratio of normalized gene expression value in NO-treated cells to value in untreated Th17 cells. RNA isolation and qPCR mRNA was isolated 48, 72 and 96 h after Th17 or Th9 differentiation using the RNeasy Micro kit (Qiagen). cDNA was synthesized using 200 ng of total RNA through a reverse transcription reaction kit (Applied Biosystems). qPCR was performed with the SYBR Green Gene Expression Assay using the ABI Prism 7,900 Sequence Detection System instrument (Applied Biosystems) according to the manufacturer’s protocol. Target gene expression was calculated using the comparative method for relative quantification after normalization to Hprt gene expression. The sequences for primers are as follows: Hprt : forward, 5′-GCAGTACAGCCCCAAAATGG-3′, reverse, 5′-AACAAAGTCTGGCCTGTATCCAA-3′; Il9 : forward, 5′-CTGATGATTGTACCACACCGTGC-3′, reverse, 5′- GCCTTTGCATCTCTGTCTTCTGG-3′; Il4ra : forward, 5′-GAGTGAGTGGAGTCCTAGCATC-3′, reverse, 5′-GCTGAAGTAACAGAACAGGC-3′; Il2 : forward, 5′-CCTGAGCAGGATGGAGAATTACA-3′, reverse, 5′-TCCAGAACATGCCGCAGAG-3′; TgfbrII : forward, 5′-CCGCTGCATATCGTCCTGTG-3′, reverse, 5′-AGTGGATGGATGGTCCTATTACA-3′; Sfpi1 : forward, 5′-GATGGAGAAGCTGATGGCTTGG-3′, reverse, 5′-TTCTTCACCTCGCCTGTCTTGC-3′. In some experiments, Nos3 and Mucin5A expression in the lungs of WT and Nos2 −/− mice immunized with OVA and challenged with OVA or PBS (described above) were analysed by qPCR. Total RNA from the lungs was extracted using Trizol reagent and analysed with the SYBR green method as above. Primers sequences are: Gapdh : forward 5-GGGTGTGAACCACGAGAAAT-3′, reverse 5′-CCTTCCACAATGCCAAAGTT-3′; Mucin5A : forward 5′-AAAGACATAGTCACTCAGCAA-3′, reverse 5′-CTGGGAAGTTCAGTGTCAAACCA-3′; Nos3 : forward 5′-GGGAAAGCTGCAGGTATTTGAT-3′, reverse 5′ CACTGTGATGGCTGAACGAAGA-3′. Enzyme-linked immunosorbent assay ELISA was carried out with paired antibodies according to the manufacturer’s instructions: mouse IL-17A, IL-9, IL-2 and human IL-9 (all from BD Biosciences). The sensitivity was <50 pg ml −1 . For the Mdm2-p53 assay, ELISA kit (Enzo Life Sciences) was used according to the manufacturer’s instruction. Murine IL-9 assay was also performed using a mouse Single-plex Cytokine Detection System (Bio-Rad) according to the manufacturer’s instructions. The plates were analysed on a Bio-Rad Bio-Plex Luminex 100 plate reader. Statistical analysis Statistical analyses were performed using GraphPad Prism 5.0. Comparisons between two groups were performed using a two-tailed unpaired Student’s t -test. Multiple groups were compared using a two-way analysis of variance followed by a Bonferroni’s post test. Values for all measurements are expressed as mean±s.e.m., P <0.05 was considered statistically significant. All experiments were performed at least two times. How to cite this article: Niedbala, W. et al. Nitric oxide enhances Th9 cell differentiation and airway inflammation. Nat. Commun. 5:4575 doi: 10.1038/ncomms5575 (2014).